Saturable absorption of intense hard X-rays in iron In 1913, Maurice de Broglie discovered the presence of X-ray absorption bands of silver and bromine in photographic emulsion. Over the following century, X-ray absorption spectroscopy was established as a standard basis for element analysis, and further applied to advanced investigation of the structures and electronic states of complex materials. Here we show the first observation of an X-ray-induced change of absorption spectra of the iron K-edge for 7.1-keV ultra-brilliant X-ray free-electron laser pulses with an extreme intensity of 10 20 W cm −2 . The highly excited state yields a shift of the absorption edge and an increase of transparency by a factor of 10 with an improvement of the phase front of the transmitted X-rays. This finding, the saturable absorption of hard X-rays, opens a promising path for future innovations of X-ray science by enabling novel attosecond active optics, such as lasing and dynamical spatiotemporal control of X-rays. Saturable absorption (SA), which denotes the decrease of absorption for higher-intensity light, is one of the typical nonlinear optical responses of matter. In the visible light region, SA was first observed in the 1940s [1] . This discovery of SA preceded the invention of lasers and is now an important factor in advanced laser technologies. One of the notable applications is an ultrafast optical modulation in the laser oscillator to generate an ultra-short pulse laser by using larger transparency at the higher intensity [2] . A beneficial feature of this simple scheme is its wide applicability to shorter wavelengths [3] , [4] from extreme ultraviolet to hard X-rays. We present potential applications of SA. First, SA enables us to control and tailor the temporal profiles of ultrafast X-ray pulses. Although X-ray free-electron laser (XFEL) sources [5] , [6] , [7] , [8] , [9] have successfully produced brilliant, femtosecond X-rays pulses, further reduction or compression of pulse duration with advanced X-ray optics has not yet been achieved. The ultrafast time response of SA provides a promising technique for generating intense attosecond X-ray pulses. Next, SA relates closely to creation of a novel non-equilibrium medium, which enables us to realize various nonlinear X-ray applications. A good example is the hollow atom solid, in which almost every atom in the solid has only one K-shell electron without disordering the atom position. Furthermore, SA in crystalline objects including heavy atoms can enhance the contrast in a multiple anomalous dispersion method and facilitate phasing under high-intensity conditions [10] . So far, SA induced by short-wavelength light has been observed for the Sn N-edge ( hν =24 eV) [4] and the Al L-edge ( hν =92 eV) [3] by using brilliant FEL [5] , [6] in the extreme ultraviolet-to-soft X-ray regions with intensities of 10 14 and 10 16 W cm −2 , respectively. Generation of SA in the hard X-ray region, however, is extremely challenging. In fact, since the Maurice de Broglie’s discovery of X-ray absorption bands in 1913 (refs 11 , 12 ), the X-ray absorption process, which widely applied for element, chemical and structural analysis of complex materials [13] , [14] , has been appropriately described by one-photon approximation at a low-intensity condition. Observing SA requires enhancing the population of atoms remaining in the excited states to a non-negligible level, so that the atoms are pumped from the ground states with photoabsorption and are unable to absorb succeeding photons. However, the lifetime of the excited states induced by hard X-rays is very short, because a core hole of the inner shell is promptly refilled by electron transition from the outer shell through Auger decay or fluorescence processes. For example, the lifetime of the K-shell core hole of Fe ( Z =26), which follows absorption of 7.1-keV X-ray quantum, is estimated to be as short as 500 as [15] . Note that this lifetime becomes shorter for higher Z atoms with higher excitation energies. One needs to use extremely intense X-ray light to achieve a large excitation rate that overcomes the decay rate. The required intensity can be roughly estimated from the photoionization rate for the cold state at the low-intensity limit, given by where μ , N atom , I and hν are the X-ray linear absorption coefficient, the number of atoms in a unit volume, the X-ray intensity and the X-ray photon energy, respectively. In the case of the K-edge of a pure iron solid, for example, the intensity I at which the photoionization rate is equal to the decay rate of 2 fs −1 is estimated to be 2 × 10 19 W cm −2 using the parameters of μ =3.2 × 10 3 cm −1 , N atom =7.8 × 10 22 cm −3 and hν =7.1 keV. This level of intensity is substantially higher than those used for recent discoveries of nonlinear optical phenomena in the soft and hard X-ray regions [16] , [17] , [18] , [19] , [20] . Although a highly efficient reflecting focusing system has been able to increase the intensity up to 10 18 W cm −2 (ref. 21 ), the intensity has still remained far below the criterion. In this article, we show the first observation of an X-ray-induced change of absorption spectra of the iron K-edge for 7.1-keV ultra-brilliant X-rays. To drastically enhance the X-ray intensity up to 10 20 W cm −2 , we used a two-stage focusing system [22] , [23] developed at SACLA [8] , [24] . For higher intensities, we successfully observed a drastic change of the absorption spectrum with an increase of transparency by a factor of 10. We also found that this bleaching effect yields a change in the far-field angular profile, which is reasonably explained by introducing an intensity-dependent complex refractive index [10] . Experimental setup The focusing system consists of a pair of focusing mirrors in the Kirkpatrick–Baez geometry. The upstream mirror system expands the XFEL beam size. The increased size of the incident beam enables us to apply a large numerical aperture to the downstream optics, which is useful for generating a very small spot with a reasonable working distance. We were able to generate a small spot with a size of 50 × 50 nm 2 , which corresponds to an extreme intensity of 10 20 W cm −2 with an X-ray pulse energy of 20 μJ and a nominal pulse duration of 7 fs. 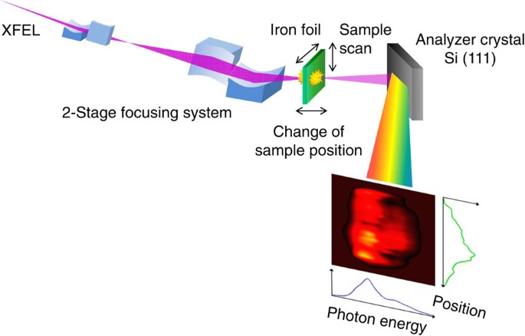Figure 1: Schematic of the experimental setup. SACLA produces 7.1-keV XFEL pulses with a bandwidth of 40 eV in full width at half maximum. The two-stage focusing system generates a small spot of 50 × 50 nm2. The spectra are recorded with a dispersive spectrometer, which consists of the final focusing system that gives a large divergence of 2.5 mrad, a flat analyzer crystal of Si and a multi-port charge coupled device detector. The intensity is controlled by changing the size of the beam on the sample, which is moved along the optical axis. Figure 1 shows a schematic of the experimental setup. For the spectral measurement, we used a dispersive crystal spectrometer [25] , [26] , which covers a wide range of spectrum (~40 eV) of the incident XFEL light generated with the Self-Amplified Spontaneous Emission scheme [27] , [28] (see Methods for details). Figure 1: Schematic of the experimental setup. SACLA produces 7.1-keV XFEL pulses with a bandwidth of 40 eV in full width at half maximum. The two-stage focusing system generates a small spot of 50 × 50 nm 2 . The spectra are recorded with a dispersive spectrometer, which consists of the final focusing system that gives a large divergence of 2.5 mrad, a flat analyzer crystal of Si and a multi-port charge coupled device detector. The intensity is controlled by changing the size of the beam on the sample, which is moved along the optical axis. 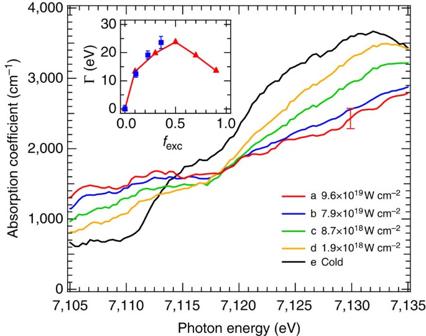Figure 2: Absorption coefficients at different X-ray intensities. Absorption coefficients for 20-μm-thick iron foil measured in the vicinity of the iron K-edge (hν=7,113 eV) at different X-ray intensities ofI=(9.6±1.1) × 1019W cm−2(a, red line), (7.9±0.9) × 1019W cm−2(b, blue line), (8.7±1.0) × 1018W cm−2(c, green line) and (1.9±0.2) × 1018W cm−2(d, yellow line), while that at the cold condition (I=(1.5±0.2) × 109W cm−2) is shown in e (black line). The error bar in a indicates a typical uncertainty due to the counting statistics. The inset shows a width Γ of the absorption edge as a function of the excitation degreefexc. The closed triangles with a line show the simulated values, while the closed squares are the experimental data. Full size image Observation of SA Figure 2 shows typical absorption spectra measured in the vicinity of the iron K-edge ( hν =7,113 eV). Here, absorption coefficients μ ( h ν) taken at different intensities are plotted as a function of photon energy. Iron foil with a thickness of 20 μm was used for the measurement. The intensity of X-rays on the foil was varied in the range of 10 18 –10 20 W cm −2 . For comparison, a cold absorption spectrum obtained at a low-intensity condition of I =(1.5±0.2) × 10 9 W cm −2 , achieved with strong attenuation, is also shown in Fig. 2 . Here we found that X-ray absorption in the spectral range above the K-edge decreases as the X-ray intensity increases. For the highest intensity condition of I =(9.6±1.1) × 10 19 W cm −2 , the absorption coefficient decreases from 3,600±110 to 2,400±140 cm −1 at h ν=7,130 eV, which corresponds to an enhancement of transmission by a factor of 10.3 for the 20-μm foil. We note that the absorbed energy density estimated from this reduction factor is much higher than 10 11 J m −3 , which is a standard criterion for the high-energy density state. Figure 2: Absorption coefficients at different X-ray intensities. Absorption coefficients for 20-μm-thick iron foil measured in the vicinity of the iron K-edge ( hν =7,113 eV) at different X-ray intensities of I =(9.6±1.1) × 10 19 W cm −2 (a, red line), (7.9±0.9) × 10 19 W cm −2 (b, blue line), (8.7±1.0) × 10 18 W cm −2 (c, green line) and (1.9±0.2) × 10 18 W cm −2 (d, yellow line), while that at the cold condition ( I =(1.5±0.2) × 10 9 W cm −2 ) is shown in e (black line). The error bar in a indicates a typical uncertainty due to the counting statistics. The inset shows a width Γ of the absorption edge as a function of the excitation degree f exc . The closed triangles with a line show the simulated values, while the closed squares are the experimental data. Full size image In Fig. 3 , the relative increase of transmission at hν =7,130 eV was plotted as a function of intensity. The intensity dependence relates closely to the decay dynamics of the excited states. To analyse the results, we performed a numerical simulation, taking into consideration the electrons in the K-shell, the L-shell and the vacuum levels. We also assumed that the rates of the Auger decay and the fluorescence processes are proportional to the number of the L-shell electrons and the K-shell vacancies. Under these assumptions, we calculated a spatiotemporal evolution of the absorption coefficient along the beam axis so as to determine the transmission. When we use a decay time of 500 as for the K-shell core hole in ref. 15 , the calculated threshold of SA is higher than the threshold measured, as seen in Fig. 3 . We can compensate for this discrepancy if we assume an elongated decay time of 2 fs, as shown in the figure. This deviation could be explained by influences of the intense resonant field of X-rays. The presence of strong Kα emission may change the fluorescence decay rate and the total decay rate, as can be observed in optical media interacting with intense visible light [29] . Another possibility is modification of the configurations of the L-shell electrons in the absorption processes. Note that this effect can be mitigated by utilizing higher photon energy above the K-absorption edge, which suppresses influences of L-shell modifications. In addition, the larger discrepancies in the intermediate intensity region ( I ~10 18 W cm −2 ) could be explained by a possible inhomogeneity in the intensity profile at the defocused condition. 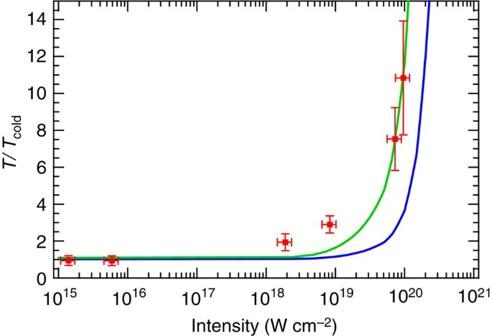Figure 3: Relative increase in transmission. TransmissionT, normalized at the cold conditionTcold, is plotted as a function of intensity athν=7,130 eV for 20-μm-thick iron foil. The square dots show the experimental results, while the blue and the green lines are simulated curves with core-hole lifetimes of 500 as and 2 fs, respectively. Figure 3: Relative increase in transmission. Transmission T , normalized at the cold condition T cold , is plotted as a function of intensity at hν =7,130 eV for 20-μm-thick iron foil. The square dots show the experimental results, while the blue and the green lines are simulated curves with core-hole lifetimes of 500 as and 2 fs, respectively. Full size image Analysis of change of absorption spectrum The change of the absorption spectrum in Fig. 2 shows a characteristic feature: as the intensity increases, we observed a decrease of absorption above the K-edge, while we found that absorption below the K-edge increases. As a result, the absorption edge becomes blurred for higher intensities. This behaviour reflects the fact that high-density excitation of 1s electrons modifies the energy levels of the remaining, unexcited 1s electrons in solids. The change in the energy level was simulated with a localized core-hole model, in which we considered the site dependence of local electrostatic potentials originating from various geometrical configurations of core-hole sites in neighbouring atoms. Using the unrestricted Hartree–Fock method, we calculated absorption spectra for different excitation degrees (for details, see the subsection ‘Change of absorption spectrum at high intensity condition’ in the Supplementary Methods ; Supplementary Figs 1–4 ). We plotted the dependence of the edge-broadening Γ on the excitation degree in the inset of Fig. 2 . We also determined the dependence of the shift of the central position Δ of the edge, as seen in Supplementary Fig. 5 . We found good agreement between the experiments and the simulations. In contrast, we found that a delocalized hole model, which is used for explaining SA in the longer wavelength excitation in the valence band [4] , imposed a blue shift of the absorption edge without any broadening (Δ>0, Γ≈0). These results did not agree with our experimental observations. Thus, as a first step, we could say that the localized core-hole approximation is more suitable for describing SA of hard X-rays. Improvement of wave front under SA We found that transparency becomes remarkably enhanced for the high-intensity region. It is interesting to investigate whether this bleaching effect could change the wave front of the transmitted beam. 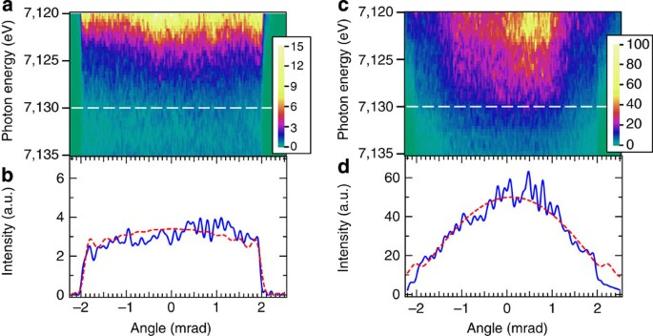Figure 4: Angular-resolved transmission spectra. Angular-resolved transmission spectra (a,c) measured at two different intensities ofI=(1.8±0.2) × 1018W cm−2(a) and (9.5±1.1) × 1019W cm−2(c). Angular profiles athν=7,130 eV along the white dashed lines ina,care shown as the solid lines in (b,d), respectively. The dashed lines inb,dare the simulated results. Figure 4a,c displays dependencies of the far-field angular profiles on photon energy for two intensity conditions, measured with the spectrometer. From these figures, we extracted the angular profiles at a photon energy of 7,130 eV, shown as solid lines in Fig. 4b,d . For the low-intensity condition at I =(1.8±0.2) × 10 18 W cm −2 , the profile shows a quasi-rectangular shape that has hard edges with a divergence of 4.0 mrad, which is consistent with the nearly flat-top profile of the incident X-ray beam to the final mirrors. In contrast, the divergence decreases to 3.0 mrad with a smooth Gaussian-like profile for the high-intensity condition at I =(9.5±1.1) × 10 19 W cm −2 . To investigate the trigger for this drastic change, we introduced an intensity-dependent complex refractive index [15] , which spatially varies in the absorption medium as a function of intensity. We then simulated the amplitude and phase of the wave fields on the exit surface of the medium (for details, see the subsection ‘Change of angular profile at high intensity condition’ in the Supplementary Methods ; Supplementary Figs 6–8 ). By combining the results with a wave-optical simulation based on Fresnel–Kirchhoff’s diffraction, we determined the angular profiles at the far-field condition, as shown by the dashed lines in Fig. 4b,d . We found an excellent agreement between the results for the simulation and the experiment. This is the first observation of intensity-driven dynamical spatial control of X-rays with improvement of the phase front. Figure 4: Angular-resolved transmission spectra. Angular-resolved transmission spectra ( a , c ) measured at two different intensities of I =(1.8±0.2) × 10 18 W cm −2 ( a ) and (9.5±1.1) × 10 19 W cm −2 ( c ). Angular profiles at hν =7,130 eV along the white dashed lines in a , c are shown as the solid lines in ( b , d ), respectively. The dashed lines in b , d are the simulated results. Full size image We discuss the potential applicability of SA for dynamical temporal control of ultrafast X-ray pulses. Using a simulation, the rise time of SA, which is proportional to the intensity, is estimated to be 1.7 fs at the maximum intensity in this experiment. This abrupt increase of transmission is useful for reducing the temporal duration of the incident pulse to the attosecond region with an appropriate control of the intensity. Our simulation shows that one could produce a 0.9-fs pulse duration by introducing a 6-fs X-ray pulse with an intensity of I =1.1 × 10 21 W cm −2 onto an 80-μm-thick iron foil (for details, see the subsection ‘Generation of attosecond X-ray pulse with SA’ in the Supplementary Methods ; Supplementary Fig. 9 ). One of the key challenges is to utilize incident X-ray pulses with a well-defined temporal profile. Although the current Self-Amplified Spontaneous Emission scheme configuration generates X-ray pulses with uncontrolled spikes, seeded XFEL technologies [9] , [30] are capable of generating single-mode pulses with high reproducibility. SA will play an important role as a link between state-of-the-art light sources and advanced optical technologies and will drive the development of X-ray science under extreme conditions. Experimental details To increase X-ray intensity, we employed a two-stage focusing system [22] , consisting of two sets of reflecting mirrors in the Kirkpatrick–Baez geometry. The first set of focusing optics enlarges the beam size at the second set of mirrors, ~70 m away. This configuration enables us to increase the numerical aperture of the second focusing system, which effectively generates a small focal spot while maintaining a large distance between the mirror and the sample. The size of the focused beam was measured by scanning a knife-edge with an application of attenuators. Divergence angles after the second set of mirrors are 2.5 mrad (horizontal) and 4.0 mrad (vertical). The iron foil was irradiated by the X-ray beam with a normal incidence condition. To avoid influences from radiation damage, we used a fresh part of the sample during the measurements. We achieved this by scanning the sample in every shot along the horizontal and vertical directions with a 50-μm step. For measuring the spectra, we used a dispersive spectrometer [26] consisting of an analyzer flat crystal of silicon (111) and a multi-port charge coupled device detector [31] . The spectral range Δ E of a dispersive spectrometer using Bragg reflection is described by Here, E , θ B and Δ θ are the photon energy, the Bragg angle and the divergence angle, respectively. The spectral range was evaluated to be 60 eV with parameters of E =7.12 keV, θ B =16.1 degrees and Δ θ =2.5 mrad. The spectral resolution Δε / E is described by Here, σ is the X-ray source size corresponding to the focal spot size, L is the distance from the source to the detector (3.7 m) and ω is the full width at half maximum of the Darwin curve for the Bragg diffraction for π -polarization. The spectral resolution was evaluated to be 800 meV. To investigate intensity dependencies, intensity must be controlled over several orders of magnitude. To accomplish this, we adjusted the size of the beam on the foil by translating the foil along the beam axis. Also, the pulse energy of the incident X-rays for every single shot was monitored using a back-scattering beam monitor [32] . To derive the profiles shown in Figs 2 and 3 , single-shot spectra measured with and without the foil were sorted by the intensity. The averages of the spectra over 100 shots in each condition were used for normalization. The error bars in Fig. 3 correspond to the s.d. How to cite this article: Yoneda, H. et al. Saturable absorption of intense hard X-rays in iron. Nat. Commun. 5:5080 doi: 10.1038/ncomms6080 (2014).